Sharply autofocused ring-Airy beams transforming into non-linear intense light bullets Controlling the propagation of intense optical wavepackets in transparent media is not a trivial task. During propagation, low- and high-order non-linear effects, including the Kerr effect, multiphoton absorption and ionization, lead to an uncontrolled complex reshaping of the optical wavepacket that involves pulse splitting, refocusing cycles in space and significant variations of the focus. Here we demonstrate both numerically and experimentally that intense, abruptly autofocusing beams in the form of accelerating ring-Airy beams are able to reshape into non-linear intense light-bullet wavepackets propagating over extended distances, while their positioning in space is extremely well defined. These unique wavepackets can offer significant advantages in numerous fields such as the generation of high harmonics and attosecond physics or the precise micro-engineering of materials. Finite-energy Airy beams were first introduced in the field of optics in 2007 (refs 1 , 2 ) as new non-diffracting wavepackets in one and two spatial dimensions. The Airy function, describing the spatial electric field profile of these beams, is the only non-spreading one-dimensional (1D) solution of the Schrödinger equation discovered in the field of quantum mechanics in 1976 (ref. 3 ). The most notable feature of the linear Airy beam is the transverse acceleration, which causes the beam to propagate in a parabolic trajectory [4] , while keeping a constant central lobe diameter. This exotic behaviour is forced by a strong spatial cubic phase which is imprinted on the beam profile. This spatial chirp causes a constant energy flux from the oscillating tail of the beam towards the main lobe, effectively forcing the beam to accelerate in the transverse direction. In addition, the Airy beam proves very resilient to perturbations, as it is able to linearly reconstruct (self-heal) itself [5] . Further research activity on Airy beams in the non-linear regime has revealed stationary non-linear 1D solutions [6] , (3+1)D non-linear light bullets [7] , solitons in self-defocusing media [8] and other newly observed spatial mechanisms [9] , [10] . Recently, the Airy wavepacket concept has also been demonstrated for electron packets [11] . The cylindrically symmetric Airy beam (or ring-Airy beam), which is able to abruptly autofocus in the linear regime, was introduced theoretically [12] and was demonstrated experimentally [13] to be able to deliver high-energy pulses inside thick transparent samples without damaging the material before the focus. The abrupt intensity increase at the focus of the ring-Airy makes it easy to combine a long working distance with a small focal volume. The remarkable abilities of the ring-Airy beam make it an ideal candidate for laser ablation applications in previously hard-to-reach environments. Here we demonstrate that the non-linear dynamics of high-power ring-Airy wavepackets are even more impressive. Using numerical simulations, we compare the attributes of high-power ring-Airy wavepackets to those of Gaussian beams carrying the same power and identify a number of exciting features, which are very useful for practical applications [14] , [15] , [16] , [17] . These include a minor non-linear focal shift and the reshaping of the wavepacket into an intense non-linear dynamic light bullet structure. In addition, we elucidate the physical origin of these interesting features by correlating them to the typical ring-Airy spatiotemporal reshaping mechanism in the focus. Finally, our theoretical findings are confirmed by experiments in bulk fused silica. Non-linear ring-Airy beams To explore the non-linear propagation dynamics of ring-Airy beams, we compare them with Gaussian beams. We consider two types of Gaussian beams that can be deemed equivalent to a given ring-Airy beam [13] , the equivalent envelope Gaussian beam (EEGB) defined as the Gaussian beam with full-width at half maximum (FWHM) equal to the diameter of the ring-Airy beam and the equivalent peak contrast Gaussian beam (ECGB), which, in the linear regime, reaches the same peak intensity contrast value at the focus (more details can be found in the beam description of the Methods section). The term peak contrast refers [12] to the ratio of the peak intensity in the beam focus to the peak intensity at the beam origin. In our simulations, both beams are focused at the focus of the ring-Airy using a lens. Both of them carry the same power; thus, the EEGB and the ECGB only differ by their beam width and initial peak intensity. Regardless of the spatial profile of the beams used, the temporal profile in our simulations was in all cases Gaussian with a FWHM of 200 fs at a central wavelength of 800 nm. Additional information about the description of the simulated wavepackets and the numerical model used in the simulations can be found in the Methods section. Focus shift in the non-linear regime We performed numerical experiments by increasing the input power for all three beams. As expected, the focus is shifted towards the laser source as the input power is increased. 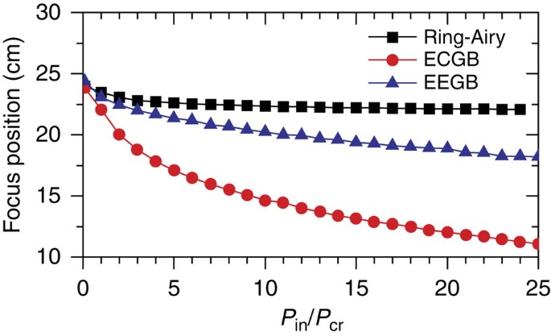Figure 1: Focus shift in the non-linear regime. Focus position as a function of the input power for the ring-Airy beam (black squares) and the two Gaussian beams with equivalent contrast (red dots) and equivalent envelope (blue triangles). Figure 1 shows a comparison of the position of the non-linear focus of the ring-Airy beam with those obtained for the two Gaussian beams. Interestingly, in the non-linear regime, the ring-Airy beam focus shift is significantly smaller compared with the two Gaussian beams as the beam power increases. For the ring-Airy, the focus position moves from 24 cm to roughly 22 cm, whereas the input power is gradually increased up to 10 P cr ( P cr being the critical power for self-focusing, see Methods for exact definition). Further increase in power, up to 24 P cr , seems to have a negligible effect on the focus position. For both Gaussian beams, the focus shift is much larger compared with the ring-Airy case. Especially for the ECGB, the focus position is shifted down to 11 cm for 24 P cr , which is more than half the initial distance. For the EEGB, the focus shift is not as strong, but still reaches 6 cm, that is, about three times more than for the ring-Airy case. The difference between the two Gaussian beams is explained by the wider beam width for the EEGB and the fact that the non-linear focus position is proportional to the Rayleigh length, that is, scales as ( w 0 2 ) [18] , [19] . In the Discussion section below, we provide an analytical approach for calculating precisely the small focus shift of the ring-Airy beams. Figure 1: Focus shift in the non-linear regime. Focus position as a function of the input power for the ring-Airy beam (black squares) and the two Gaussian beams with equivalent contrast (red dots) and equivalent envelope (blue triangles). Full size image Spatial dynamics and filament formation The peak intensity of the ring-Airy beam is shown in Fig. 2a as a function of the propagation distance for five different input powers. As the input power is increased, the distribution of the peak intensity along the beam propagation changes significantly, showing an escalating abrupt increase near the focus. For example, at 5 P cr , the first peak appears much more abruptly and the consecutive secondary peaks, although spatially separated in the linear regime, merge into an almost uniform filament sustaining high peak intensities over a longer propagation distance, compared with the linear case (black continuous line). As the power is gradually increased and non-linearities come into play, the secondary peaks gradually merge and rise in intensity until the formation of a continuous intensity plateau at P in >10 P cr . At these powers, the peak intensity is almost constant ≅ 2.5 × 10 13 W cm −2 along the plateau, without significantly increasing as the input power is further increased. This can be understood in terms of intensity clamping [20] due to the presence of non-linear losses, which are strong enough to limit the increase of the peak intensity. The resulting structure is a long filament similar to filaments obtained by propagation of high-power Gaussian beams [18] , except that it results from the collapse of a ring-Airy beam as detailed below. This is clearly demonstrated in Fig. 2b , where the peak intensity of a ring-Airy beam at the plateau region ( z =40 cm) is shown in comparison with two Gaussian beams as a function of the input power. The peak intensity for all beams is practically identical for input powers above 5 P cr . A graphic representation of the transformation of a ring-Airy beam, where the discrete sharp intensity peaks in the linear regime transform into a uniform filament in the non-linear regime, is shown in Fig. 2c . 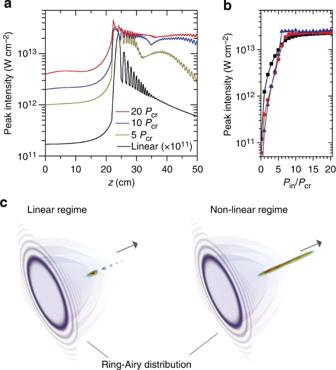Figure 2: Simulation results in the non-linear propagation regime in air. (a) Peak intensity distribution of the ring-Airy beam versus propagation distance for various input powers. (b) Maximum peak intensity at the plateau region (z=40 cm) as a function of the input power for the ring-Airy (black squares), EEGB (blue triangles) and ECGB (red dots). (c) Graphic representation of accelerating ring-Airy beams in the linear and non-linear regime. Figure 2: Simulation results in the non-linear propagation regime in air. ( a ) Peak intensity distribution of the ring-Airy beam versus propagation distance for various input powers. ( b ) Maximum peak intensity at the plateau region ( z =40 cm) as a function of the input power for the ring-Airy (black squares), EEGB (blue triangles) and ECGB (red dots). ( c ) Graphic representation of accelerating ring-Airy beams in the linear and non-linear regime. Full size image Spatiotemporal effects and light bullet formation Besides the minor focal shift and the formation of a filament, interesting spatiotemporal dynamics take place beyond the focal region. 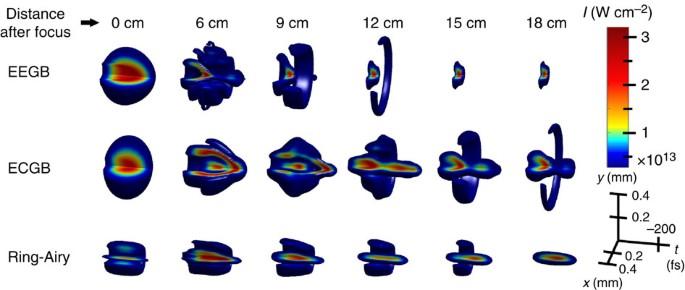Figure 3: Spatiotemporal dynamics in the non-linear propagation regime. Intensity isosurfaces for an EEGB (first row), an ECGB (second row) and a ring-Airy wavepacket (third row) at various positions alongzafter the non-linear focus. Beam propagation direction is from left to right. Figure 3 depicts the intensity isosurfaces for an EEGB (first row), an ECGB (second row) and a ring-Airy wavepacket (third row) for various propagation distances beyond the non-linear focus. Figure 3: Spatiotemporal dynamics in the non-linear propagation regime. Intensity isosurfaces for an EEGB (first row), an ECGB (second row) and a ring-Airy wavepacket (third row) at various positions along z after the non-linear focus. Beam propagation direction is from left to right. Full size image Each of the three wavepackets carries ten critical powers. Because of the different non-linear dynamics ( Fig. 1 ), the actual focus position (denoted as 0 cm in Fig. 3 ) along the propagation axis is different for each beam. The two Gaussian beams exhibit a typical severe spatiotemporal reshaping process extensively studied in the literature [18] , [21] . As shown in Fig. 3 , the initial Gaussian wavepacket is reshaped into a ring structure with an intense spot that is split in the temporal domain. We can clearly see that for both cases the space and time distributions of the wavepacket are constantly evolving in a complex way, as expected in filamentation of Gaussian beams. The dynamic reshaping action of non-linear effects diminishes after ∼ 15 cm. After this point, both Gaussian wavepackets spread owing to linear diffraction and dispersion. On the other hand, the spatiotemporal dynamics of the ring-Airy beam are very different. The wavepacket has the form of a ring with an intense core in its centre, whereas no pulse splitting is obtained in the temporal domain. This non-linear light-bullet structure propagates without significant changes over 15 cm. Only after 18 cm of propagation, the non-linear dynamics start to weaken and the ring-Airy wavepacket starts to spread due to the action of diffraction and dispersion. The annular structure that surrounds the ring-Airy intense peak at 15 cm after the focus, although resembles a similar annular feature formed in the Gaussian wavepacket, is generated by different mechanisms. In the case of the non-linear ring-Airy beam, the ring is sustained by the combination of the pre-organized energy flux from the tail to the main lobe of the Airy profile [12] , [13] and light coming from the non-linear focus, diffracted by the generated plasma. In the case of the Gaussian beam, the ring is generated by a spontaneous transformation of the Gaussian beam into a Bessel-like beam induced by non-linear effects [22] and featured by conical emission [23] . This type of non-linear ring formation depends on the multiphoton order of the non-linear absorption and is discussed in details in the case of two-photon absorption in ref. 24 . Experimental demonstration To confirm the validity of the simulation findings, we performed non-linear propagation experiments of ring-Airy beams in fused silica. The use of fused silica is beneficial both in terms of the energy needed ( P cr is much lower than air) and also in the visualization of the non-linear propagation by exploiting the accompanying two-photon red fluorescence emission [25] . Detailed information about the experimental procedure and the analysis used to estimate the intensity profile of the ring-Airy beam can be found in the Methods section. Typical non-linear fluorescence emission images are shown in Fig. 4a . It is clearly visible that the non-linear focus shifts as the input energy is increased. Furthermore, low-intensity secondary peaks, characteristic to the ring-Airy, are emerging after the primary focus. The experimentally measured intensity distribution along the propagation axis I (0, z ) for various ring-Airy input energies is depicted in Fig. 4b . 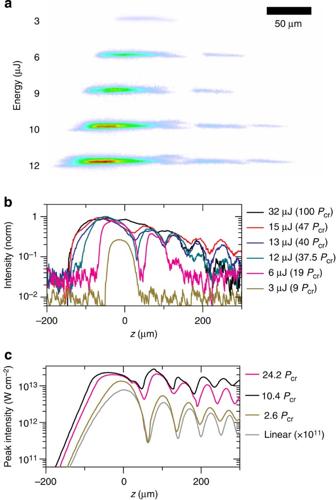Figure 4: Experimental and simulation results of the non-linear propagation regime in the bulk of fused silica. (a) Non-linear fluorescence emission images in false colours (the beam propagates from left to right). (b) Experimental intensity distribution (normalized values) along the propagation axis for various input energies. The curves are shifted upwards for visualization purposes. (c) Comparative numerical simulation results of the peak intensity along the propagation. Figure 4: Experimental and simulation results of the non-linear propagation regime in the bulk of fused silica. ( a ) Non-linear fluorescence emission images in false colours (the beam propagates from left to right). ( b ) Experimental intensity distribution (normalized values) along the propagation axis for various input energies. The curves are shifted upwards for visualization purposes. ( c ) Comparative numerical simulation results of the peak intensity along the propagation. Full size image As predicted by the theoretical simulations in the non-linear propagation regime, the consecutive peak contrast is reduced as the beam energy is increased. At high-enough energies, the intensity maxima are merged to a single intense filament along the propagation axis. This trend is verified in Fig. 4c by numerical simulations we performed in fused silica for the same input parameters as in the experiments. One may also note in both experiments and simulations the gradual decrease of the focus shift with increasing input energy as with the simulations in air above. An important question to answer for the purpose of predicting the position of the focus in a given experimental situation (as the one shown in Fig. 2a ) is what is the mechanism leading to the small non-linear focus shift for the ring-Airy, and, even more importantly, can a scaling law be derived? As the spatial profile of the ring-Airy beam is significantly different from that of a typical Gaussian beam, the well-known Marburger’s formula [19] cannot be used to predict the collapse distance. The collapse of a ring-Airy beam can be described in two stages: (i) a quasi-linear stage, during which the ring structure shrinks over a propagation distance f min and follows a parabolic trajectory (see Methods section, equation (4)); (ii) a second stage from f min to the collapse distance f rAi , during which the intensity of the ring-Airy beam increases more abruptly and the assumption of a quasi-1D trajectory for the peak intensity no longer holds. This happens when the primary ring reaches a sufficiently small diameter to induce significant mutual attraction between opposite parts of the ring, in analogy with the mutual attraction and merging of two individual filaments induced by cross Kerr effects when they are separated by less than approximately three typical filament diameters [26] . Pursuing this analogy, we assume that in the case of ring-Airy beams as well, non-linear effects will take over when the diameter of the primary ring is ∼ 3 times that of the diameter of a typical filament in the medium. Using equation (4) from the Methods section, we can estimate the propagation distance f min from the condition R ( f min )=3 w α /2: where w α ≅ 90 μm is the typical filament diameter in air and R 0 ∼ 980 μm. In our case, the ring-Airy focus in the linear regime is f =23.95 cm. For the second stage, a simple empirical formula that fits nicely the simulation results for the non-linear focus shift as a function of the ring-Airy input power P in is given by: where P cr refers to the critical power [19] of a Gaussian beam with the same central wavelength and γ ≡ P Ring / P in is a scaling parameter referring to the fraction of power contained in the primary ring of the ring-Airy distribution. The quantity f−f min corresponds to the maximum shift that can be reached at very large powers, where the optical Kerr effect abruptly focuses on the primary ring. A comparison of the focus shift estimated by our numerical simulations and the prediction of the empirical formula of equation (2) is shown in Fig. 5a . 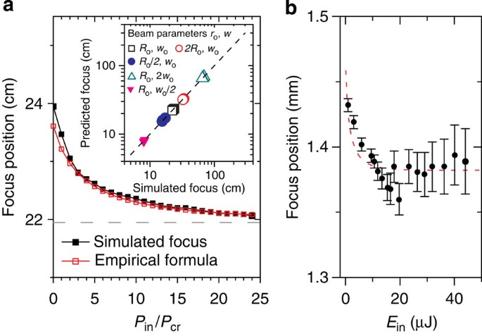Figure 5: Simulations and experiments on the non-linear focus shift. (a) Focus shift for the ring-Airy as a function of the input power for propagation in air. Simulation results (black dots), empirical formula (red line),fminempirical limiting focus position (gray dashed line). Inset: comparison between expected and simulated focus position (the mean error is 1%, whereas the maximal error is 3%). (b) Experimentally measured focus shift in fused silica. (Error bars denote s.d., the dotted red curve is the empirical formula prediction). Figure 5: Simulations and experiments on the non-linear focus shift. ( a ) Focus shift for the ring-Airy as a function of the input power for propagation in air. Simulation results (black dots), empirical formula (red line), f min empirical limiting focus position (gray dashed line). Inset: comparison between expected and simulated focus position (the mean error is 1%, whereas the maximal error is 3%). ( b ) Experimentally measured focus shift in fused silica. (Error bars denote s.d., the dotted red curve is the empirical formula prediction). Full size image To confirm that equation (2) adequately predicts the non-linear focus position for different ring-Airy beams, we have performed simulations for a range of ring-Airy beam parameters (different radii and widths). The predicted and simulated focus position for various ring-Airy beams is shown in the inset of Fig. 5a . In all cases, equation (2) clearly predicts the focus position of the ring-Airy beam. To further validate equation (2) we compare its prediction in Fig. 5b , against the measured focus shift as a function of the input energy for the experimentally generated ring-Airy beam in fused silica (see Fig. 4a ). Again, although the propagation medium is now different, the theoretical prediction using equation (2) clearly fits the experimental findings. In conclusion, ring-Airy wavepackets present unique features in the non-linear regime. The non-linear focus shift, as the beam power is increased, is much smaller for a ring-Airy beam compared with equivalent Gaussian beams and can be precisely predicted with a simple semi-empirical formula we derived considering the Kerr-induced ring collapse. Although, the most exciting feature is that beyond the focal region, the otherwise localized, in the linear regime, ring-Airy wavepacket is reshaped into an intense non-linear light bullet. Finally, we have also offered the first experimental demonstration of these predictions performing experiments in fused silica. The level of control achieved with these wavepackets offers unique advantages for applications that require regulated paths of high intensities, such as harmonic generation, laser micromachining and remote sensing. Beam description Three different laser beam profiles were used in the simulations, a ring-Airy beam and two Gaussian beams. All simulations were done in air at atmospheric pressure. The ring-Airy beam electric field [13] is described by the following equation: where Ai () corresponds to the Airy function [3] , r is the radial coordinate, r 0 represents the radius of the primary ring, α is a truncation constant and w is a scaling factor. More precisely, the primary ring of the beam has its peak intensity at a radius of R 0 ≡ r 0 – w · g ( α ), where g(α) denotes the first zero of the function Ai′( x )+ α ·Ai( x ), whereas its FWHM is ∼ 2.28 w (ref. 13 ). The power content carried by the beam is numerically calculated by integration of the starting spatial intensity profile over the whole computational box (5 mm radius). The linear focus of the ring-Airy beam can be analytically described by the beam parameters , by considering large ring-Airy beams as quasi-1D structures, that is, the trajectory of the intensity maximum of the ring-Airy beam in the linear regime is given by the quadratic acceleration for the 1D Airy beams [1] , [13] : In our simulations, we used r 0 =921 μm, w= 61.4 μm and α= 0.05, leading to g(α) ∼ −0.97. Using these parameters, the ring-Airy beam is autofocusing at a position z =23.95 cm. The widths at 1/ e 2 radius of the EEGB and ECGB are 1,738 and 855 μm, respectively. 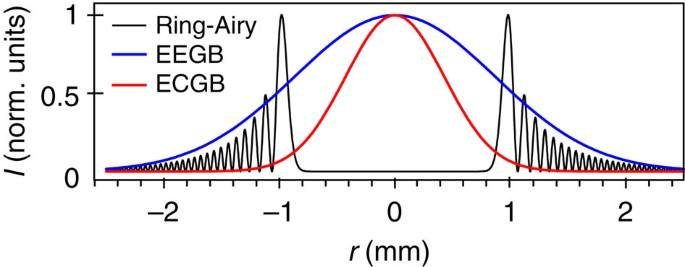Figure 6: Comparative plot of intensity distributions. Radial intensity distribution of the ring-Airy, EEGB and ECGB used in the simulations. Figure 6 shows the radial intensity distribution of the ring-Airy and both Gaussian beams. Figure 6: Comparative plot of intensity distributions. Radial intensity distribution of the ring-Airy, EEGB and ECGB used in the simulations. Full size image Numerical model The numerical model [18] that is used in the simulations resolves a non-linear envelope equation governing the propagation along the z direction of the pulse envelope E(r,z,t) in cylindrical coordinates. It takes the form of a canonical unidirectional propagation equation in the generalized few-cycle envelope approximation [21] , [27] and reads in the Fourier domain: the first (linear) term on the right-hand side includes the effects of diffraction, dispersion and space–time coupling: , where and the dispersive properties of the medium are described by a Sellmeier relation k (ω) for air [28] , and denote the carrier wavenumber at the central frequency ω 0 , the linear refractive index in air at ω 0 and . The non-linear dispersion function describes the self-steepening operator where the non-linear polarization represents the optical Kerr effect, c is the speed of light in vacuum and ɛ 0 is the vacuum permittivity. The derivation is explained in details in ref. 21 . The non-linear terms in equation (1) are all included in the non-linear polarization envelope and current envelope , which are calculated in the space–time ( τ,r,z) domain, where denotes time in the local pulse frame. The non-linear polarization describes the optical Kerr effect: where the coefficient for the Kerr non-linearity in air n 2 =3.2 × 10 −19 cm 2 W −1 leads to a critical power for self-focusing ∼ 3.2 GW. The current describes plasma absorption and plasma defocusing in the framework of the Drude model, with collision time τ c : where ρ denotes the density of the plasma generated by multiphoton ionization and avalanche. The various parameters in equations (6) and (7) are the cross section for inverse Bremsstrahlung =5.5 × 10 −20 cm 2 calculated from the Drude model with the collision time τ c =350 fs in air, the cross section for multiphoton absorption β K = Kħ ω 0 ρ nt σ K =4 × 10 −95 cm 13 W −7 , and σ K =3.4 × 10 −96 cm 16 W −8 s −1 denotes the coefficient for multiphoton ionization with K =8 photons at 800 nm for ionizing oxygen molecules with an initial density ρ nt =0.5 × 10 18 cm −3 . Equation (5) is coupled with an evolution of equation (8) for the electron density, which describes plasma generation by multiphoton ionization with rate W MPI = σ K I K and avalanche: U i =12.03 eV denotes the ionization potential of oxygen molecules. Experimental implementation As shown in Fig. 7 , we used 160 fs, 800 nm laser pulses, with a Gaussian spatiotemporal distribution, produced by a 50-Hz Ti:Sapphire laser system. To generate the ring-Airy beam, we followed a Fourier transform approach described in detail in ref. 13 . In brief, the method is based on modulating the phase of a Gaussian beam (using a Hamamatsu LCOS-X10468-2 phase reflecting only spatial light modulator), which is then Fourier transformed by a lens. The ring-Airy distribution is then generated in the Fourier transform plane of the lens after blocking the zero-order diffraction. To further reduce the effective focal length of the generated ring-Airy beam, we reduced its transverse size by ∼ 17 times, using a 4f optical system composed by a 300-mm lens and a × 8 (0.2 numerical aperture) microscope objective. 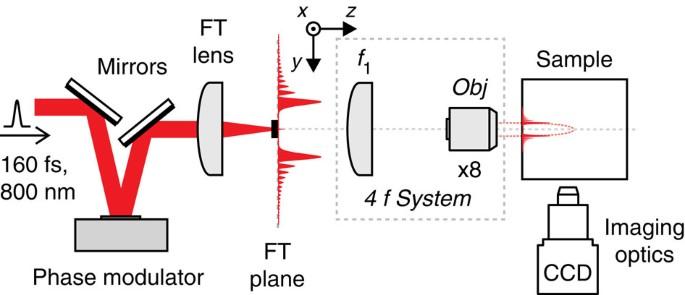Figure 7: Experimental setup. FT, Fourier transform. FT lens (400 mm);f1(300 mm); Obj (microscope objective × 8, 0.2 numerical aperture). Figure 7: Experimental setup. FT, Fourier transform. FT lens (400 mm); f 1 (300 mm); Obj (microscope objective × 8, 0.2 numerical aperture). Full size image The red fluorescence emission, induced by the high intensity of the ring-Airy beam in the focus region, was imaged using a compact microscope system (0.2 numerical aperture) and a linear charge-coupled device camera (12 bit, 1,224 × 968 pixels). Using the fluorescence emission images, we were able to estimate the intensity distribution of the propagating beam. More specifically, the observed fluorescence is actually an Abel transform of a radially symmetric fluorescence emission in the focal volume. By applying inverse Abel transform on the images, we estimate the radial distribution of the fluorescence emission F ( r,z ). The beam intensity I ( r,z ) distribution can be then extracted from F ( r,z ) I 2 ( r,z ). Although this method does not provide an absolute estimation of the beam intensity, it can be used to accurately estimate its spatial distribution. How to cite this article: Panagiotopoulos, P. et al. Sharply autofocused ring-Airy beams transforming into non-linear intense light bullets. Nat. Commun. 4:2622 doi: 10.1038/ncomms3622 (2013).